Tensile testing of ultra-thin films on water surface The surface of water provides an excellent environment for gliding movement, in both nature and modern technology, from surface living animals such as the water strider, to Langmuir–Blodgett films. The high surface tension of water keeps the contacting objects afloat, and its low viscosity enables almost frictionless sliding on the surface. Here we utilize the water surface as a nearly ideal underlying support for free-standing ultra-thin films and develop a novel tensile testing method for the precise measurement of mechanical properties of the films. In this method, namely, the pseudo free-standing tensile test, all specimen preparation and testing procedures are performed on the water surface, resulting in easy handling and almost frictionless sliding without specimen damage or substrate effects. We further utilize van der Waals adhesion for the damage-free gripping of an ultra-thin film specimen. Our approach can potentially be used to explore the mechanical properties of emerging two-dimensional materials. The surface of water has a high surface tension of 73 mN m −1 due to the strong intermolecular hydrogen bonding [1] between water molecules. To break its surface requires a large force, and this enables contacting objects to remain afloat. Furthermore, almost frictionless sliding on the water surface is possible due to its low viscosity, only 1.002 mPa s −1 at room temperature [2] . We adopt these superior characteristics of the water surface to develop a pseudo free-standing tensile testing method for ultra-thin films. This is intended to overcome the limitations of existing tensile tests for thin films, such as difficulties in the fabrication and handling of free-standing specimens without damage, or the accurate extraction of mechanical properties from the tensile tests of supported thin films. The mechanical properties of thin films, such as Young’s modulus, yield strength, tensile strength and ductility, have been of paramount importance to many thin film applications, including microelectronic, biological technologies and energy conversion devices [3] , [4] , [5] . They are generally measured by tensile testing of either free-standing thin films without substrates [6] , [7] , [8] , [9] or supported thin films on compliant substrates [10] , [11] , [12] . The free-standing tensile test is able to measure the mechanical properties of thin films directly without cumbersome calculation from substrate effects. Nevertheless, the free-standing tensile test has disadvantages, in particular with fabricating and handling of free-standing thin-film specimens without damage, resulting from difficulties in separating the specimen from the substrate, and subsequent manipulation without forming wrinkles and cracks [8] . In contrast, the supported thin-film tensile test is also widely used as an alternative method, owing to advantages of convenient specimen fabrication and handling, by utilizing an underlying compliant substrate. This method codeforms a thin film with a polymer substrate to obtain composite film/substrate stress–strain data, from which the mechanical properties of the thin film can be extracted [10] . However, when the film thickness is critically smaller than the substrate thickness, the extraction becomes challenging because of the difficulty in distinguishing a diminutive force exerted in the thin film from the relatively gigantic force applied to the film/substrate composite. The aforementioned drawbacks of the two types of thin-film tensile tests are expected to worsen with decreasing film thickness, such as sub-100 nm ultra-thin films. In this work, we develop a pseudo free-standing tensile test utilizing the characteristics of water to eliminate the drawbacks and exploit the advantages of both the free-standing tensile tests and supported tensile tests. As shown in Figs 1b , 2b–f and 3 , specimen preparation and tensile testing procedures are performed on the surface of either water or water-diluted etchant solution, to achieve a damage-free specimen afloat on the water surface that can glide frictionless during the pseudo free-standing tensile test. The advantages of water surfaces have been also utilized in the electrochemical synthesis of nanoporous Au thin films [13] . Furthermore, a gripping method using polymer-coated grips is devised to attach loading grips to the thin-film specimen by van der Waals adhesion. A digital image correlation (DIC) device is set up for real-time strain measurement [14] , [15] . In the end, we have been able to apply tensile force to the floated specimens and directly measure stress–strain curves, from which the mechanical properties of ultra-thin films can be obtained. 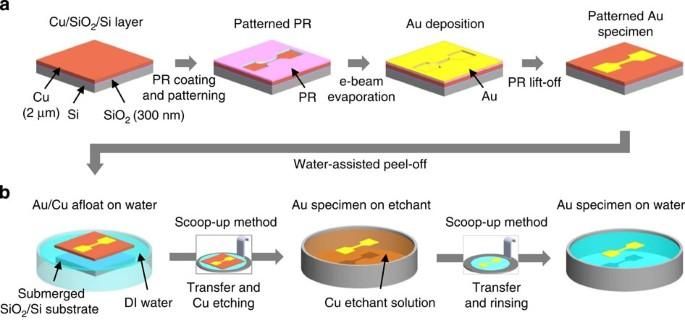Figure 1: Schematic illustration of the specimen fabrication and transfer processes. (a) Fabrication of a dog-bone-shaped Au thin film specimen. Two-μm-thick Cu is evaporated as a sacrificial substrate on a thermally grown 300-nm-thick silicon dioxide (SiO2) layer. Photo resist (PR) is patterned using a Cr mask and Au is deposited by an electron-beam evaporator. The Au specimen on a Cu/SiO2/Si substrate is patterned by PR lift-off. (b) Processes for releasing the Au specimen onto deionized (DI) water surface using water-assisted mechanical peel-off and Cu wet etching. The Cu layer is removed by water-diluted iron chloride (FeCl3) etchant, and the Au specimen remaining on the surface of the etchant is transferred onto the water surface using a scoop-up method. Figure 1: Schematic illustration of the specimen fabrication and transfer processes. ( a ) Fabrication of a dog-bone-shaped Au thin film specimen. Two-μm-thick Cu is evaporated as a sacrificial substrate on a thermally grown 300-nm-thick silicon dioxide (SiO 2 ) layer. Photo resist (PR) is patterned using a Cr mask and Au is deposited by an electron-beam evaporator. The Au specimen on a Cu/SiO 2 /Si substrate is patterned by PR lift-off. ( b ) Processes for releasing the Au specimen onto deionized (DI) water surface using water-assisted mechanical peel-off and Cu wet etching. The Cu layer is removed by water-diluted iron chloride (FeCl 3 ) etchant, and the Au specimen remaining on the surface of the etchant is transferred onto the water surface using a scoop-up method. 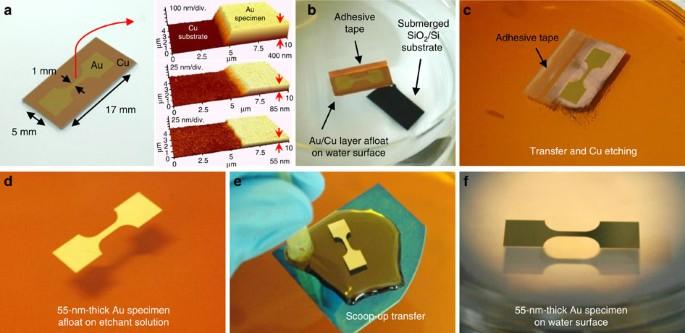Figure 2: Transfer processes for the tensile test specimen. (a) Au specimens fabricated on Cu/SiO2/Si substrate, with various thicknesses of 400, 85 and 55 nm measured by atomic force microscopy. (b) Peel-off process between the Au/Cu layer and the SiO2/Si substrate is performed on the water surface using an adhesive tape with water assistance, resulting in the Au/Cu layer afloat on the water surface. (c) The Au/Cu layer is transferred from the water surface to the surface of etching solution (FeCl3) using the scoop-up method and the Cu layer is removed. (d) The ultra-thin Au film specimen afloat on the etchant solution after Cu etching. (e) The scoop-up method for specimen transfer. (f) The ultra-thin Au specimen transferred on water surface. Full size image Figure 2: Transfer processes for the tensile test specimen. ( a ) Au specimens fabricated on Cu/SiO 2 /Si substrate, with various thicknesses of 400, 85 and 55 nm measured by atomic force microscopy. ( b ) Peel-off process between the Au/Cu layer and the SiO 2 /Si substrate is performed on the water surface using an adhesive tape with water assistance, resulting in the Au/Cu layer afloat on the water surface. ( c ) The Au/Cu layer is transferred from the water surface to the surface of etching solution (FeCl 3 ) using the scoop-up method and the Cu layer is removed. ( d ) The ultra-thin Au film specimen afloat on the etchant solution after Cu etching. ( e ) The scoop-up method for specimen transfer. ( f ) The ultra-thin Au specimen transferred on water surface. 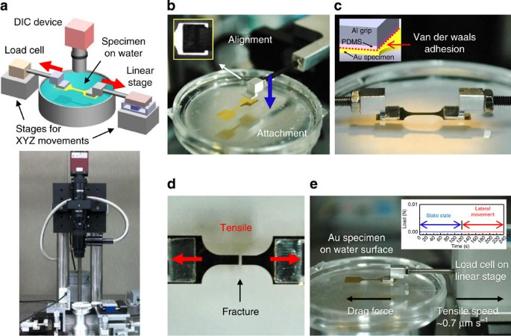Figure 3: Tensile testing procedures and the effect of drag force. (a) The tensile testing system consists of a load cell, a linear stage and a DIC camera on an anti-vibration table. (b) The ultra-thin Au film afloat on the water surface with alignment and grip attachment. Specimen gripping is performed by attaching PDMS-coated grips to the specimen’s grip sections. Meanwhile, alignment is ensured through the DIC camera. (c) The ultra-thin Au film specimen is strongly gripped by van der Waals adhesion between the PDMS coating on the grips and the specimen surface. (d) Tensile test is performed by linear stage with the strain rate of 0.06 × 10−3per s, and fracture occurred in the middle of the specimen’s gauge length. (e) Drag force measurement has been made by attaching only one side of the specimen to the load cell connected to the linear stage. Full size image Figure 3: Tensile testing procedures and the effect of drag force. ( a ) The tensile testing system consists of a load cell, a linear stage and a DIC camera on an anti-vibration table. ( b ) The ultra-thin Au film afloat on the water surface with alignment and grip attachment. Specimen gripping is performed by attaching PDMS-coated grips to the specimen’s grip sections. Meanwhile, alignment is ensured through the DIC camera. ( c ) The ultra-thin Au film specimen is strongly gripped by van der Waals adhesion between the PDMS coating on the grips and the specimen surface. ( d ) Tensile test is performed by linear stage with the strain rate of 0.06 × 10 − 3 per s, and fracture occurred in the middle of the specimen’s gauge length. ( e ) Drag force measurement has been made by attaching only one side of the specimen to the load cell connected to the linear stage. Full size image Fabrication and transfer of ultra-thin film specimens The fabrication, peel-off, etching and transfer processes for the thin-film specimen are shown in Fig. 1 . A dog-bone-shaped Au specimen was fabricated on a Cu/SiO 2 /Si substrate by photo-resist patterning and lift-off processes ( Fig. 1a ). Through subsequent water-assisted peel-off and Cu-etching processes, the specimen for the tensile test was transferred onto the water surface by a scoop-up method ( Fig. 1b ). To begin with, gold was selected as the material for the tensile test specimen, because it is the least reactive metal towards atoms or molecules at the interface with a gas or a liquid [16] . Therefore, the effect of any possible chemical reaction at the interface between the Au specimen and underlying water can be neglected. Moreover, the mechanical behaviour of free-standing Au thin films with thickness above 100 nm has been widely studied [15] , [17] , [18] , [19] , [20] , [21] , which is useful for the validation of our tensile testing method. However, to the best of our knowledge, ultra-thin Au films with thickness below 100 nm have not been tested by the free-standing tensile test due to the difficulties in the specimen fabrication and handling without damage. Au specimens with various thicknesses of 400, 85 and 55 nm were fabricated on the Cu/SiO 2 /Si substrate ( Fig. 2a ). A 2-μm-thick Cu film deposited by electron beam evaporation on a SiO 2 /Si substrate was used as a sacrificial layer to enable the subsequent water-assisted peel-off ( Fig. 2b ) and the release of the Au specimen onto the surface of the etchant solution through Cu wet etching ( Fig. 2c,d ). Because of poor adhesion between Cu and SiO 2 , the Au/Cu layer can be easily peeled off from the SiO 2 /Si substrate. Carrying out this process on a water surface leads to the Au/Cu layer afloat on the water surface ( Fig. 2b ). Adhesive tape is used to make an initial crack between Cu and SiO 2 . Through a scoop-up method, the Au/Cu layer is transferred from the water surface to the surface of the etchant solution. Water-diluted iron chloride (FeCl 3 ) solution (CE-100, Transene Company Inc.) was used as an oxidizing etchant and this removes the Cu substrate efficiently without forming gaseous products or precipitates ( Fig. 2c ). After Cu etching, the ultra-thin Au film specimen is subsequently left floating on the etching solution ( Fig. 2d ). The specimen on the etching solution is scooped up ( Fig. 2e ), and transferred to the water surface ( Fig. 2f ). Tensile testing procedures on water surface The tensile testing system for the ultra-thin film specimen on water surface is shown in Fig. 3a (see Methods). Although the specimen is afloat on the water surface in a static state, polydimethylsiloxane (PDMS)-coated grips are attached to specific sections for gripping the specimen ( Fig. 3b ). Meanwhile, the alignment of the specimen is arranged by the charge-coupled device (CCD) camera’s image ( Fig. 3b , inset). Our specimen-gripping technique utilizes van der Waals adhesion between the 5-μm-thick PDMS coating on the grips and the specimen surface, resulting in easy manipulation and strong gripping force for tensile testing the ultra-thin films, without slippage or delamination ( Fig. 3c , inset, and also see Supplementary Note 1 ). It does not require any adhesive bonding, external electrostatic force or mechanical fastening, and therefore provides convenient gripping of the ultra-thin film specimen ( Fig. 3c ). The tensile test is performed with a strain rate of ~6.0 × 10 −5 per s through the linear stage until the final fracture of the specimen occurs ( Fig. 3d ). For measurement of the strain through the DIC device, finely ground graphite particles were deposited as displacement marks at the ends of the specimen gauge length. During the tensile test, the load and strain data are directly measured by the load cell and the DIC device independently. For the validation of the testing procedures, the van der Waals adhesion for the gripping technique, the specimen alignment and possible bending moment exerted on the specimen are carefully investigated. We have selected the PDMS for a gripping material because of its superior adhesion to the solid surfaces without slippage or delamination during the tensile test (see Supplementary Note 1 for the validation details). Regarding the specimen alignment, the coordination of pixels from the CCD camera’s images and XYZ positioning microstages are used for the in-plane alignment; the out-of plane alignment is ensured by the intensity of the brightness within the error of ~2 μm (see Supplementary Note 2 ). Finally, as for the possible bending moment effects and consequent errors of the tensile stress on the specimen, the finite element analysis showed the possible errors from the eccentric loading are negligible (see Supplementary Note 3 and Supplementary Movies 1–6 ). The effect of frictional drag force To ensure the pseudo free-standing state for the floating specimen, first the liquid surface should keep the thin-film specimen afloat. Second, the frictional drag force caused by the liquid surface should be negligible. Therefore, the selection criteria for the supporting liquid are high surface tension, low viscosity and non-reactivity to the specimen (see Supplementary Note 4 ). Various liquids such as water, hydrogen peroxide, methanol and acetone are considered; only water perfectly satisfies the selection criteria. Possible frictional drag force exerted on the sliding specimen by the water surface was directly investigated. One side of the specimen was attached to the PDMS-coated grip and the load cell combined with the linear stage was moved for 120 s with the speed of ~0.7 μm s −1 , which is the speed for the tensile test ( Fig. 3e ). During the static state before movement of the linear stage, the load data shows noise with maximum amplitude less than ~60 μN, which is only 0.27% of the breaking load for 55 nm films. Measured load data during movement of the specimen also shows the same data from the static state ( Fig. 3e , inset). This reveals the drag force caused by the water surface is almost negligible compared with the breaking load of the 400-, 85- and 55-nm-thick Au film specimens, which were ~0.2, 0.034 and 0.022 N, respectively. Accordingly, we can conclude that the water surface hardly affects the specimen and apparently provides a pseudo free-standing state for ultra-thin films, without frictional drag force or any other substrate effects. Using our tensile testing method for ultra-thin films, the mechanical properties of ultra-thin Au film specimens were successfully measured. Stress–strain curves for the tested films and their fractured surfaces are shown in Fig. 4 . When film thickness decreases from 400 to 55 nm, the average value of Young’s modulus and ductility decrease from 67±4 to 55±4 GPa and 2.0% to 0.9%, respectively ( Fig. 4a–c ). Each value represents the average of three specimens tested. The results of the tensile tests show the strong thickness dependence of the mechanical behaviour of the thin films. The measured Young’s modulus of the 400-nm-thick specimen is consistent with the previous reported value of ~68 GPa measured by another existing method [17] . For the thin films with thickness below 100 nm, we were able to obtain reduced values, 58±4 and 55±4 GPa for 85- and 55-nm-thick specimens, respectively. In particular, the stress–strain curve shows linear elastic behaviour up to fracture with small plasticity as the film thickness decreases [18] . The reduction of modulus can be attributed to the anelastic behaviour [22] , film density [23] and grain boundary compliance [7] , [24] . As the film thickness goes to ultra-thin scale with smaller grain size, the grain boundary region occupies the significant part of the film [25] , and it becomes elastically softer than the grain interior resulting in the reduced modulus [19] , [26] . The fractured surfaces of each specimen were characterized by scanning electron microscope as shown in Fig. 4d–i . The images of the fractured surface of the 400-nm-thick specimen show clear necking as a result of ductile fracture ( Fig. 4d,e ). In contrast, brittle fracture with significantly reduced ductility is observed for the ultra-thin films below 100 nm ( Fig. 4f–i ). 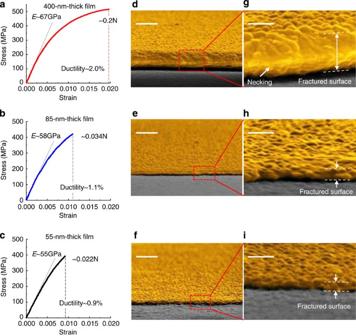Figure 4: Mechanical properties and failure analysis of the tensile test specimens. (a–c) Stress–strain curves of the 400-, 85- and 55-nm-thick Au film specimens. As the thickness of the Au specimen decreases, Young’s modulus and ductility decrease. (d) Scale bar, 500 nm, (e) scale bar, 200 nm, (f) scale bar, 500 nm, (g) scale bar, 200 nm, (h) scale bar, 500 nm, (i) scale bar, 200 nm. Scanning electron microscopy images of the fractured surface of the 400-, 85- and 55-nm-thick film specimens. Figure 4: Mechanical properties and failure analysis of the tensile test specimens. ( a – c ) Stress–strain curves of the 400-, 85- and 55-nm-thick Au film specimens. As the thickness of the Au specimen decreases, Young’s modulus and ductility decrease. ( d ) Scale bar, 500 nm, ( e ) scale bar, 200 nm, ( f ) scale bar, 500 nm, ( g ) scale bar, 200 nm, ( h ) scale bar, 500 nm, ( i ) scale bar, 200 nm. Scanning electron microscopy images of the fractured surface of the 400-, 85- and 55-nm-thick film specimens. Full size image As mentioned above, our result for the 400-nm-thick specimen is almost same with the one measured by other existing method, which demonstrates the validity of our method. Regarding the Au thin films with thickness below 100 nm, there is only one previously reported study [27] by the supported tensile test that can be referred, to the best of our knowledge. However, the measured mechanical properties of the 100-nm-thick Au films from the supported tensile test varied significantly depending on the type of the polymer substrate employed due to the substrate effect: the elastic modulus and the ductility were 367 GPa and ~4% on the polysulphone substrate, and 271 GPa and ~7.5% on the 4,4′-(1-hydroxyphenylidene) diphenol substrate. Moreover, the ductility of ~4.5% from the Au/polysulphone for the 50-nm-thick Au films are significantly overvalued, which are mainly provided by compliant substrate [28] , [29] . In our method, on the other hand, the tensile testing of ultra-thin Au film on water surface was accomplished accurately without the substrate effect. In conclusion, we have developed the pseudo free-standing tensile testing system and used it to investigate the mechanical properties of ultra-thin Au films. Our method utilizes the superior characteristics of the water surface, which has high surface tension and low viscosity, enabling damage-free fabrication, easy handling of thin-film specimens afloat on the water surface, with negligible frictional drag force. A novel gripping technique using van der Waals adhesion between PDMS and the specimen is utilized for the damage-free gripping of the ultra-thin film specimens. We were able to directly measure the mechanical properties of ultra-thin Au films using our method. The results showed the reduced modulus and ductility from 67 to 55 GPa and 2.0% to 0.9%, respectively, with decreasing thickness from 400 to 55 nm. Adopting the water surface and van der Waals adhesion, we overcame not only the challenging fabrication and handling of ultra-thin film specimens from free-standing tensile test but also the limitations regarding substrate effects and loading extraction from supported tensile test. This will open up new possibilities to explore various ultra-thin and two-dimensional materials such as graphene [30] , [31] , ultra-thin Si [32] , metal oxides [33] and organic-inorganic hybrids [34] , as well as biomembranes [5] , essentially in contact with a liquid surface. Tensile testing system The pseudo free-standing tensile testing system consists of a load cell, a linear stage and a DIC device on an anti-vibration table. The tensile force is measured by load cells (LTS-50GA and 10GA, KYOWA, Japan). An ultra-high resolution linear DC motor (M-111.1 DG, PI, Germany) with a controller (C-863, PI, Germany) is used for linear displacement. Micro XYZ positioning stages are placed under the load cell and the linear stage for specimen alignment. The DIC device is set up using a CCD camera (F-145Bs IRF, Marlin, Germany) with a microscope and this ensures the continuous observation of the specimen with real-time strain monitoring. All devices and data acquisition are directly controlled by the LabVIEW programme (National Instruments, USA). How to cite this article: Kim, J. -H. et al . Tensile testing of ultra-thin films on water surface. Nat. Commun. 4:2520 doi: 10.1038/ncomms3520 (2013).